Steric engineering of metal-halide perovskites with tunable optical band gaps Owing to their high energy-conversion efficiency and inexpensive fabrication routes, solar cells based on metal-organic halide perovskites have rapidly gained prominence as a disruptive technology. An attractive feature of perovskite absorbers is the possibility of tailoring their properties by changing the elemental composition through the chemical precursors. In this context, rational in silico design represents a powerful tool for mapping the vast materials landscape and accelerating discovery. Here we show that the optical band gap of metal-halide perovskites, a key design parameter for solar cells, strongly correlates with a simple structural feature, the largest metal–halide–metal bond angle. Using this descriptor we suggest continuous tunability of the optical gap from the mid-infrared to the visible. Precise band gap engineering is achieved by controlling the bond angles through the steric size of the molecular cation. On the basis of these design principles we predict novel low-gap perovskites for optimum photovoltaic efficiency, and we demonstrate the concept of band gap modulation by synthesising and characterising novel mixed-cation perovskites. Hybrid organic–inorganic perovskites [1] , [2] , [3] , [4] recently surged to worldwide attention following the report of highly efficient solar cells based on methylammonium lead halides [5] , [6] , [7] , [8] . In fact, within less than 2 years of development, the photovoltaic energy-conversion efficiency of these devices increased from the initial 10.9% (ref. 5 ) to the current record of 17.9% (NREL certified) and 19.3% (uncertified) [9] . This impressive trend fuelled the expectation that perovskite photovoltaics may soon revolutionize the solar energy landscape. Given the unusually long lifetimes of the photoexcited carriers [10] , [11] , [12] and the relatively low optical gap [13] , [14] , it has been proposed that the perovskite layer may act both as the light absorber and as the electron and hole transporter [15] , similarly to bulk semiconductor solar cells. Within this scenario, it is expected that the energy-conversion efficiency can be increased by following the standard Schockley–Queisser analysis, that is by reducing the optical band gap to values near 1.3–1.4 eV (ref. 16 ). Substantial efforts are currently underway to optimize these solar cells by modifying the metal–halide network or the organic cation [13] , [14] , [17] , [18] , [19] , [20] , [21] , [22] , [23] . A major challenge in this research area is that, on the experimental front, the structural, electronic and optical properties of metal-organic perovskites are very sensitive to processing conditions. Similarly, computational modelling studies appear sensitive to the level of theory and calculation details. This state of affairs suggests that it may be convenient to shift the focus from the investigation of a few prototypical perovskites to global searches relying on rational design approaches. In this work we propose that, instead of modifying the metal–halide network as already conducted in refs 13 , 14 , it could be advantageous to start from MA-PbI 3 (MA=CH 3 NH 3 ) and modify its electronic and optical properties without altering the PbI 3 network. This strategy would allow us to investigate potential improvements while retaining highly desirable features such as long carrier lifetimes [10] , [12] . In the following, using a combination of geometric arguments and first-principles calculations, we demonstrate that it should indeed be possible to modulate the optical gap of lead-iodide perovskites over almost an electronvolt by acting on the Pb–I–Pb bond angles in the PbI 3 network. These angles, in turn, can be tailored using cations of different sizes, without altering the metal–halide chemistry. Platonic model of metal-halide perovskites MA-PbI 3 belongs to the family of perovskites of chemical formula ABX 3 . The simplest possible ABX 3 perovskite consists of a high-symmetry cubic structure belonging to the space group , as shown in Fig. 1a (ref. 24 ). In this structure the halogen atoms X=I occupy the vertices of regular corner-sharing BX 6 octahedra, while the divalent metal atoms B=Pb sit at the centres of the octahedra. The smallest volume enclosed by neighbouring octahedra defines a cuboctahedral cavity and hosts the monovalent cation A=CH 3 NH 3 . All the other possible perovskite structures can be imagined as obtained by rotating or distorting the BX 6 octahedra, displacing the B metal atoms off-centre and rotating the A cations within the cuboctahedral cavity [24] . 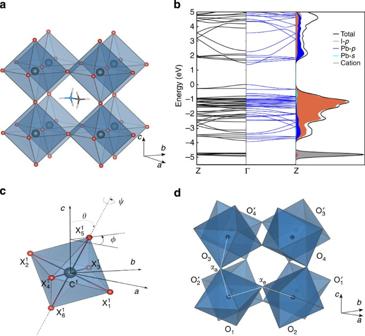Figure 1: Platonic model of metal–halide perovskites. (a) Ball-and-stick representation of MA–PbI3in the high-temperature cubic phase: the dark spheres inside the octahedra represent Pb atoms, the red spheres at the octahedral corners are I atoms and the molecule inside the cuboctahedral cavity is CH3NH3. (b) DFT scalar-relativistic electronic band structure and partial density of states of MA–PbI3in the low-temperature orthorombic phase. In the band structure plot we compare the electronic structure of MA–PbI3with (left) or without (right) the cation. The density of states shows that the electronic states associated with the cation are located far from the band gap. The top of the valence band is derived from I-5pstates and, to a smaller extent, the Pb-6sstates. The bottom of the conduction band is derived primarily from Pb-6pand I-5pstates. The calculated band gap is direct at Γ. (c) Schematic representation of the Euler angles defining the rotation of the Platonic octahedron: tilt (θ), spinningand precession (φ). The convention for labelling the corners of the octahedron is indicated, together with the crystallographic axes. (d) Schematic representation of the orthorhombic unit cell considered in this work consisting of four inequivalent octahedra, O1–O4(dark blue) and their periodic replicas(light blue). The labelling of the corners follows the same convention indicated inc. The intrinsic metal–halide–metal bond angles are highlighted: apical angle (αa) and equatorial angle (αe). The geometric properties of this model are derived in the Methods section. Figure 1: Platonic model of metal–halide perovskites. ( a ) Ball-and-stick representation of MA–PbI 3 in the high-temperature cubic phase: the dark spheres inside the octahedra represent Pb atoms, the red spheres at the octahedral corners are I atoms and the molecule inside the cuboctahedral cavity is CH 3 NH 3 . ( b ) DFT scalar-relativistic electronic band structure and partial density of states of MA–PbI 3 in the low-temperature orthorombic phase. In the band structure plot we compare the electronic structure of MA–PbI 3 with (left) or without (right) the cation. The density of states shows that the electronic states associated with the cation are located far from the band gap. The top of the valence band is derived from I-5 p states and, to a smaller extent, the Pb-6 s states. The bottom of the conduction band is derived primarily from Pb-6 p and I-5 p states. The calculated band gap is direct at Γ. ( c ) Schematic representation of the Euler angles defining the rotation of the Platonic octahedron: tilt ( θ ), spinning and precession ( φ ). The convention for labelling the corners of the octahedron is indicated, together with the crystallographic axes. ( d ) Schematic representation of the orthorhombic unit cell considered in this work consisting of four inequivalent octahedra, O 1 –O 4 (dark blue) and their periodic replicas (light blue). The labelling of the corners follows the same convention indicated in c . The intrinsic metal–halide–metal bond angles are highlighted: apical angle ( α a ) and equatorial angle ( α e ). The geometric properties of this model are derived in the Methods section. Full size image Figure 1b shows the electronic band structure of MA-PbI 3 , which represents the starting point of our investigation. Here we see that the electronic states at the top of the valence bands are of halide p -character, while those at the bottom of the conduction band are mainly derived from the metal p states. At the same time the electronic states associated with the cation define bonding and antibonding bands arranged symmetrically around the band gap and located several electronvolts away from the band edges. An analysis of the electronic charge density shows that, as expected, the cation is singly ionized, and the PbI 3 network is negatively charged [25] , [26] , [27] . These observations suggest that the electronic structure of these metal-organic perovskites may be described by removing the cation from the structural model and compensating the negative charge of the PbI 3 network using a positive background. Figure 1b shows that the band structure obtained within this approximation is in good agreement with that from a complete calculation. The removal of the cation is especially useful since it eliminates the complications associated with the observed orientational disorder [13] , [17] , [28] , [29] . Another important observation can be made by inspecting X-ray diffraction data, as reported for example in ref. 17 . In fact, from the structural parameters reported in that work we deduce that the Pb–I bond lengths are extremely regular, the largest relative deviation from the average value of 3.18 Å being 0.1%. Furthermore, the diagonals of the PbI 6 octahedra are almost perpendicular to each other, the maximum deviation from right angles being of 4°. Therefore, to a good approximation the PbI 6 octahedra may be considered as Platonic solids carrying the full O h symmetry. On the basis of these considerations we set to build a Platonic model of metal-halide perovskites, consisting of regular corner-sharing PbI 6 octahedra and no cation, as shown in Fig. 1d . In order to construct our model we start from a single regular octahedron in an orthorhombic unit cell [17] , with one diagonal parallel to the c axis, and the four perpendicular edges parallel to the axes a and b . In the reference frame of the octahedron this diagonal and its perpendicular edges define the apical and equatorial directions, respectively. Within this model, the most general perovskite structure is obtained by three successive rotations around c , a and c again using the standard Euler angles [30] , as shown in Fig. 1c : the spinning around the apical direction, the tilt θ around the a axis and the precession φ around the c axis. After these rotations, the location and orientation of all the remaining octahedra in the orthorhombic unit cell are completely determined by the corner-sharing connectivity, the metal-halide bond length and the periodicity of the crystal structure. The details of this geometric construction are given in the Methods. An immediate result of our construction is that the only way to ensure corner-sharing connectivity is by having a vanishing spinning angle . This leaves us with only two independent angular parameters, θ and φ , which refer to a spherical system of coordinates clamped on the crystallographic unit cell. It is convenient to make a change of variables to intrinsic angular parameters that are independent on the choice of the unit cell. To this end we express θ and φ in terms of the metal-halide–metal bond angles α a and α e , as indicated in Fig. 1d . α a denotes the Pb–I–Pb bond angles along the apical direction and α e those along the equatorial direction. The relation between these intrinsic angles and the Euler angles is given in the Methods. At this point the atomic structure of the Platonic perovskite model is uniquely determined by the choice of two metal–halide–metal bond angles and the metal–halide bond length. Given that the effect of bond length variations on the electronic and optical properties of these systems has been studied in detail, both theoretically [27] and experimentally [13] , our geometric analysis clearly directs attention to the role of the two inequivalent Pb–I–Pb angles. Band gap and metal–halide–metal bond angle In Fig. 2 we show the band gap of the Platonic model calculated using density functional theory (DFT) as a function of the apical and equatorial bond angles α a and α e . For definiteness we set the Pb–I bond length to the average value measured in ref. 17 . The incomplete coverage of the parameter space in Fig. 2 reflects the fact that only certain pairs of apical and equatorial angles are compatible with the corner-sharing connectivity, as discussed in the Methods. The extremal parameters of this map are, on the one side, α a = α e =180° (bottom left corner), corresponding to the most symmetric cubic perovskite structure with collinear Pb–I–Pb bonds. On the other side we have α a = α e =120° (top right corner), which we have been chosen by considering a limiting structure where the shortest distance between iodine atoms belonging to different octahedra matches the I 2 bond length ( α a =0 and α e =126°). 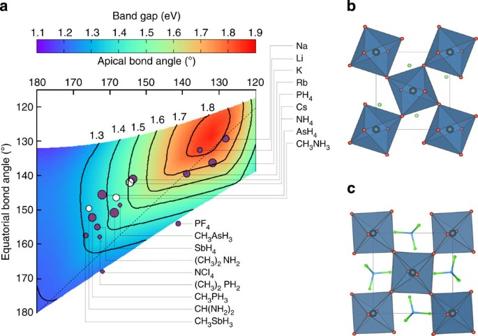Figure 2: Mapping the band gap landscape of metal-halide perovskites. (a) Two-dimensional map of the DFT band gap of the Platonic model of PbI3-based perovskites as a function of the apical and equatorial metal–halide–metal bond angles. The Pb–I bond length is set to the experimental value for MA-PbI3(ref.17). The anglesαaandαeare indicated inFig. 1d. The calculations for the Platonic model were performed within scalar-relativistic DFT (fully relativistic calculations are shown inFig. 3b, see Methods). The dashed line at 45° is a guide to the eye and shows the approximate symmetry of the map with respect the the exchange of the apical and equatorial angles. The dark discs represent the angular coordinates (αa,αe) of realistic models of PbI3-based perovskites including the cation (indicated by the chemical formula), with structures fully optimized within DFT. The apical and equatorial angles are the averages among all the inequivalent angles of the same type. The size of each circle represents the deviation of the Pb–I bond length from that of MA–PbI3(3.18 Å). This quantity is displayed because the metal–halide bond length has a small but non-negligible effect on the band gap, which we quantify as a linear shift of ~3 eV/Å (refs27,31). For the same angular coordinates, the band gap difference between the largest and the smallest circle in the figure is 0.2 eV. The white discs correspond to perovskites already synthesized13,17,18. This map shows that the band gap can be modulated over a much wider range than currently possible. (b,c) Atomistic models of the hypothetical metal-halide perovskites identified in this work exhibiting the smallest (LiPbI3) and the largest (NCl4PbI3) metal–halide–metal bond angles, respectively. Figure 2: Mapping the band gap landscape of metal-halide perovskites. ( a ) Two-dimensional map of the DFT band gap of the Platonic model of PbI 3 -based perovskites as a function of the apical and equatorial metal–halide–metal bond angles. The Pb–I bond length is set to the experimental value for MA-PbI 3 (ref. 17 ). The angles α a and α e are indicated in Fig. 1d . The calculations for the Platonic model were performed within scalar-relativistic DFT (fully relativistic calculations are shown in Fig. 3b , see Methods). The dashed line at 45° is a guide to the eye and shows the approximate symmetry of the map with respect the the exchange of the apical and equatorial angles. The dark discs represent the angular coordinates ( α a , α e ) of realistic models of PbI 3 -based perovskites including the cation (indicated by the chemical formula), with structures fully optimized within DFT. The apical and equatorial angles are the averages among all the inequivalent angles of the same type. The size of each circle represents the deviation of the Pb–I bond length from that of MA–PbI 3 (3.18 Å). This quantity is displayed because the metal–halide bond length has a small but non-negligible effect on the band gap, which we quantify as a linear shift of ~3 eV/Å (refs 27 , 31 ). For the same angular coordinates, the band gap difference between the largest and the smallest circle in the figure is 0.2 eV. The white discs correspond to perovskites already synthesized [13] , [17] , [18] . This map shows that the band gap can be modulated over a much wider range than currently possible. ( b , c ) Atomistic models of the hypothetical metal-halide perovskites identified in this work exhibiting the smallest (LiPbI 3 ) and the largest (NCl 4 PbI 3 ) metal–halide–metal bond angles, respectively. Full size image The variation of the angular coordinates in Fig. 2 clearly induces a substantial modulation of the band gap, from the top of the mid-infrared (1.1 eV) to the beginning of the visible spectrum (1.9 eV). This trend is in line with earlier calculations on simpler two-dimensional (2D) Sn-I perovskites for solution-processable electronics [31] . The qualitative trend shown in Fig. 2 can be interpreted using elementary tight-binding arguments. If we consider for definiteness the bottom of the conduction band at Γ, which is most affected by bond angles, in the case of α a = α e =180° there are three degenerate electronic states derived from the 6 p orbitals of Pb (without considering spin–orbit coupling for simplicity; this coupling is fully included in all our final results presented in Fig. 3b ). It is intuitive that the energy of these states results mainly from ppσ bonding integrals since all the Pb-I bonds are collinear [32] . By moving away from the bottom left corner, the degeneracy is lifted as the bond integrals acquire ppπ components weighted by the angles α a and α e . Both components tend to raise the energy levels; therefore, the conduction band bottom results from the competition between the antibonding orbitals with the lowest energy along the apical or the equatorial direction. This is consistent with the approximate symmetry of the map in Fig. 2 with respect to the line corresponding to α a = α e . More importantly, this reasoning suggests that the band gap of the Platonic perovskite model is governed by the largest Pb–I–Pb bond angle in the metal–halide network, consistent with the trend in Fig. 2 . This relation between band gap and bond angles holds unchanged when considering fully relativistic calculations including spin–orbit corrections. In fact, as shown in Supplementary Fig. 1 , relativistic effects induce a large but slowly varying red shift of 0.8–1.1 eV across the family of compounds considered in this work. For the sake of completeness we also checked that excitonic effects play only a minor role, with exciton-binding energies never exceeding 80 meV as shown by Supplementary Fig. 2 . Details on the calculation of exciton binding energies are given in the Methods, and the results are discussed in the Supplementary Note 1 . 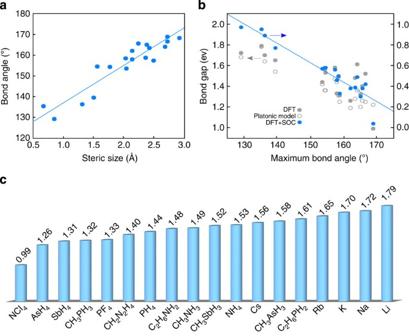Figure 3: Tuning the band gap of metal-halide perovskites via the steric size of the cation. (a) Correlation between the apical and equatorial bond angles of PbI3-based perovskites and the steric radius of the cation (discs). As the size of the cation increases the metal–halide–metal bonds (seeFig. 1d) tend to become collinear. A linear least-square fit to the data (straight line) yields a slope of 18°/Å. (b) Correlation between the DFT band gap and the largest metal–halide–metal bond angle in the structure. We show calculations for the Platonic model (circles) and fully optimized structures within scalar-relativistic (grey discs) and fully relativistic (blue discs) DFT. The arrows point to the scales corresponding to each set of data. The significant data dispersion at large angles is due to the distortions of the octahedra. The calculations based on the Platonic model include the effect of the average Pb–I bond length on the band gap, as discussed inFig. 2. (c) Calculated band gaps (in eV) of all the PbI3-based perovskites considered in this work. The band gaps were obtained after full structural optimization within scalar relativistic DFT (see Methods). Figure 3: Tuning the band gap of metal-halide perovskites via the steric size of the cation. ( a ) Correlation between the apical and equatorial bond angles of PbI 3 -based perovskites and the steric radius of the cation (discs). As the size of the cation increases the metal–halide–metal bonds (see Fig. 1d ) tend to become collinear. A linear least-square fit to the data (straight line) yields a slope of 18°/Å. ( b ) Correlation between the DFT band gap and the largest metal–halide–metal bond angle in the structure. We show calculations for the Platonic model (circles) and fully optimized structures within scalar-relativistic (grey discs) and fully relativistic (blue discs) DFT. The arrows point to the scales corresponding to each set of data. The significant data dispersion at large angles is due to the distortions of the octahedra. The calculations based on the Platonic model include the effect of the average Pb–I bond length on the band gap, as discussed in Fig. 2 . ( c ) Calculated band gaps (in eV) of all the PbI 3 -based perovskites considered in this work. The band gaps were obtained after full structural optimization within scalar relativistic DFT (see Methods). Full size image After taking into account the presence of the cation and the variations in the Pb-I bond lengths and Pb–I–Pb angles, the calculated band gaps deviate from the idealized predictions in Fig. 2 by 0.1–0.3 eV (see Fig. 3 and discussion below). Nonetheless, the general trend, which spans a range of up to 1 eV, is robust. This picture is also confirmed by relativistic GW calculations on a few selected compounds, as shown in Supplementary Fig. 4 . The trend identified here suggests that in order to make low-gap perovskites for optimum photovoltaic efficiency we need to engineer structures with minimal octahedral tilt. On the other hand, in order to make large-gap perovskites for light-emitting diodes operating in the visible, we need to design structures with maximum tilt. The remaining question is how the tilt angle can be controlled. Controlling metal–halide–metal bond angles via the steric size of the cation The Pb–I–Pb bond angles define the volume of the cuboctahedral cavity; therefore, it is intuitive that the use of larger cations may lead to values of α a and α e closer to straight angles [33] . In the search for such cations we perform DFT calculations for existing structures as well as for many hypothetical structures not considered hitherto, including full structural optimizations and spin–orbit interactions, in the presence of the cation (see Methods). In order to relate these structures and their properties to the predictions of the Platonic model, we consider the average values of the Pb–I–Pb bond angles and of the Pb–I bond length over a crystalline unit cell. These values are used as the coordinates needed for locating each structure on the map of Fig. 2 . Previously reported cations are methylammonium (ref. 17 ), formamidinium (refs 13 , 18 ), the alkali metal Cs + [18] (synthesised) and ammonium (refs 34 , 35 , 36 ) (proposed). As shown in Fig. 2 all these cations cluster around the centre of the map; therefore, they are not expected to yield a significant modulation of the band gap. In line with this result their measured optical absorption onsets are very similar, within 0.25 eV (refs 13 , 18 ). In order to explore a wider portion of the map we consider four different families of cations generated from those above. The first family consists of secondary, tertiary and quaternary ammonium cations, namely di-, tri- and tetra-methylammonium. These are large molecules obtained by replacing hydrogen atoms bonded to the N atom with methyl groups. The second family is generated from ammonium by descending the pnictogen column in the periodic table, that is by substituting N for P, As or Sb. Members of this family include phosphonium , arsonium , stibonium , and similarly the methylammonium analogues , and . The third family of cations that we consider is obtained by replacing hydrogen in ammonium by halogen atoms, and possibly nitrogen by another pnictogen: in this group we have , , , and . The fourth and final family simply consists of the alkali metals Li + , Na + , K + and Rb + . In total, we consider 22 structures, including 18 hypothetical compounds not reported to date. In order to quantify the steric size of each cation, we use the radius of the sphere that contains 95% of the DFT electron density. This choice ensures that the steric radii of the alkali metals are in agreement with their standard ionic radii [37] . For completeness the calculated steric sizes are reported in Supplementary Table 1 . Figure 3 shows that the steric radii of the cations considered in this work span a wide range, from 0.7 Å (Li + ) to . Our structural optimizations indicate that for some of the large cations the three-dimensional (3D) perovskite network is significantly distorted. This is in line with previous studies showing that large molecular cations determine a reorganization of the 3D perovskite network into a 2D layered structure [38] , [39] . These large molecules include tertiary and quaternary methylammonium cations, as well as the tetrafluoride and the tetrachloride . As these structures depart substantially from the 3D metal–halide network considered in this work, a separate analysis would be required. Accordingly, we do not consider them further. Figure 3a shows that the largest Pb–I–Pb angles correlate strongly with the steric size of the cation (Spearman correlation 88%), in line with our initial expectation. The newly proposed structures span a range of angles from 130° to 170°, thereby covering a much wider portion of the band gap map in Fig. 2 than presently possible. In addition, Fig. 3b shows that, in agreement with the predictions of the Platonic model, the band gap correlates strongly with the largest Pb–I–Pb angle in the unit cell (Spearman correlation 91%). For completeness in Fig. 3b we report the band gaps obtained from this model as well as those calculated using the fully optimized structures within fully relativistic DFT calculations. The scatter of the data, which is clearly visible in Fig. 3b , is mostly because of the variation of the Pb–I bond lengths in the metal–halide network. We calculated the correlation coefficient between band gap and bond lengths using the same data, and we obtained a very weak correlation (Spearman coefficient 9%). This test clearly indicates that the role of bond lengths represents a second-order effect, thereby providing further support to our Platonic model. Finally, Fig. 3c shows our main finding, namely that by suitably choosing the cation it is possible, at least in principle, to fine-tune the band gap almost continuously over a very wide range of photon energies. Our analysis highlights several new promising structures, in particular perovskites with phosphonium , arsonium and stibonium , all with band gaps ranging between 1.2 and 1.4 eV. These values fall in the middle of the range for optimum photovoltaic efficiency, and suggest that our new structures hold potential as novel solar cells materials. Besides the low gap, these perovskites are expected to exhibit higher mobilities than MA–PbI 3 . In fact, as shown in Supplementary Fig. 2a,b , the carrier-effective masses decrease towards larger bond angles, consistent with the concomitant reduction of the band gap. In addition to lower gaps and effective masses, large cations have the advantage that the filling of the cuboctahedral cavity should counter the known tendency of perovskite solar cells to degrade by water incorporation [14] . In order to evaluate the practical feasibility of the hypothetical perovskites identified in this work we searched for possible dynamical instabilities in one of the structures with the smallest band gap, AsH 4 PbI 3 ( is less interesting because of safety concerns related to chlorides). This structure is especially interesting since the preparation could proceed through the corresponding iodide AsH 4 I (ref. 40 ), similarly to the case of methylammonium iodide CH 3 NH 3 I. As shown by Supplementary Fig. 3 , the vibrational density of states calculated using density-functional perturbation theory [41] does not exhibit any soft modes, thereby indicating that the 3D perovskite structure of AsH 4 PbI 3 should be stable against distortions. More generally, in order to assess the stability of all the structures considered here, we move to a simple semi-empirical approach based on the Goldschmidt tolerance factor t (refs 33 , 42 ) (see Methods for the definition of t ). It is known empirically that 3D perovskites should form when the tolerance factor falls within a narrow range t =0.7–1.1 (refs 33 , 42 , 43 , 44 ). 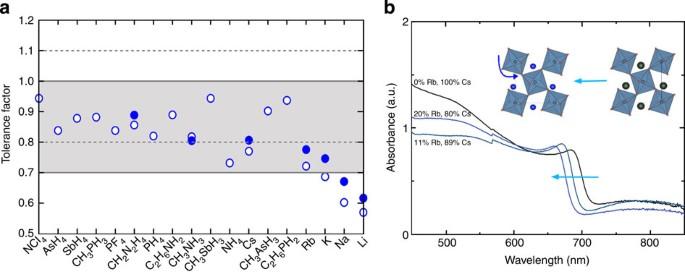Figure 4: Material stability and optical measurements. (a) Calculated Goldschmidt tolerance factors for all the perovskite structures considered in this work. The open circles are obtained using the steric sizes calculated from DFT (Supplementary Table 1). For comparison we also show the tolerance factors obtained by using the ionic radii reported in ref.37(filled circles). The grey area bound by the solid grey lines correspond to the geometric criterion for the Goldschmidt tolerance factor42,43, while the dashed lines correspond to the empirical range proposed in ref.44. (b) Measured absorbance spectra of the dark phase of RbxCs1−xPbI3perovskite thin films, withx=0,x=0.1 andx=0.2. When increasing the Rb content a continuous blue shift of the absorption onset is observed, from 720 nm (x=0) to 690 nm (x=0.2). This blue shift corresponds to an increase in band gap, and is assigned to the more pronounced octahedral tilt in the PbI3network, as illustrated in the inset. Figure 4a shows that the tolerance factors derived from our calculated steric sizes falls within this range for most of the structures considered here. In particular, according to this criterion, all the cations up to Rb and K should be stable. Figure 4: Material stability and optical measurements. ( a ) Calculated Goldschmidt tolerance factors for all the perovskite structures considered in this work. The open circles are obtained using the steric sizes calculated from DFT ( Supplementary Table 1 ). For comparison we also show the tolerance factors obtained by using the ionic radii reported in ref. 37 (filled circles). The grey area bound by the solid grey lines correspond to the geometric criterion for the Goldschmidt tolerance factor [42] , [43] , while the dashed lines correspond to the empirical range proposed in ref. 44 . ( b ) Measured absorbance spectra of the dark phase of Rb x Cs 1− x PbI 3 perovskite thin films, with x =0, x =0.1 and x =0.2. When increasing the Rb content a continuous blue shift of the absorption onset is observed, from 720 nm ( x =0) to 690 nm ( x =0.2). This blue shift corresponds to an increase in band gap, and is assigned to the more pronounced octahedral tilt in the PbI 3 network, as illustrated in the inset. Full size image In order to demonstrate the band gap tunability we attempted the synthesis of perovskites based on elemental cations, building on our experience with CsPbI 3 (ref. 18 ) (see Methods). As deposited, we observed that CsPbI 3 formed a pale phase with a wide bandgap. Upon annealing this structure turned into a dark phase with a band gap of 1.73 eV, which we identify as the 3D perovskite structure discussed in this work. The synthesis of films with cations smaller than Cs (Rb, K, Na and Li) yielded similar pale phases. However, upon annealing, some of the films degraded via sublimation before we could observe a dark phase as for CsPbI 3 , suggesting that 3D perovskites were not formed. This finding is in agreement with our analysis of the Goldschmidt tolerance factor shown in Fig. 4a . While the proposed 3D perovskites could possibly be synthesised using higher pressures or longer annealing runs at lower temperatures, here for the sake of simplicity we did not pursue this direction. Instead we considered an alternative approach and explored mixtures of cations, as suggested in ref. 45 : if mixtures of Cs and smaller cations could gradually shift the bandgap towards the larger values, this would confirm our predicted tunabiliy via steric effects. As a proof-of-concept we prepared perovskites with Rb/Cs cation mixtures, namely Rb x Cs 1− x PbI 3 with x =0, x =0.1 and x =0.2 (never hitherto reported). Optical characterization of these films, shown in Fig. 4b , indicates that the absorption edge blue shifts from 720 to 690 nm in going from Cs to Rb. This result is in excellent agreement with our calculations, which predict a corresponding blue shift of 40 nm. Our findings are also in line with a recent study (which appeared while the present manuscript was under review) where the authors demonstrated band gap tunability via the mixing of mixtures [46] . Taken together, our present results and those of refs 13 , 18 , 47 confirm the tunability of the band gap via the steric size of the cation over almost half of our predicted range, thereby providing strong support to our theory. Finally, our theory is based on very general considerations and its predictions are not linked to the underlying calculation methods. Therefore, it is expected that this model will carry similar predictive power across other families of metal–halide perovskites. More fundamentally, the ability to control the band gap via the steric size of the cation, as proposed in this work, may become a new paradigm in the solution deposition of solar cells, light-emitting diodes and photonic structures with layer-by-layer control of their optical properties. Note added in proof. While this work was under peer review, a related work exploring the relation between the size of cations and the electronic and optical properties of metal-halide perovskites was submitted and published [63] . The key difference between the present work and that of ref. 63 is that we develop a predictive universal theory of band gap tuning via steric effects, and we perform experiments that confirm a posteriori our predictions. Computational methods All calculations were performed within the local density approximation to density functional theory [48] , [49] using planewaves and pseudopotentials, as implemented in the Quantum ESPRESSO software package [50] . Only valence electrons were described explicitly, and the core–valence interaction was taken into account by means of ultrasoft pseudopotentials [51] , [52] with nonlinear core correction [53] . For Pb and I we used fully relativistic ultrasoft pseudopotentials. In the case of Pb we included the 5 d semicore states, and for Sb, Rb and Cs we used norm conserving pseudopotentials [54] . The electron wavefunctions and the charge density were expanded in planewave basis sets with kinetic energy cutoffs 40 and 200 Ry, respectively. Structural optimization was performed by sampling the Brillouin zone using uniform and unshifted 4 × 4 × 4 meshes. Electronic structure calculations were performed using a 6 × 6 × 6 Brillouin zone grid. All structural optimizations were initialized using the crystallographic data for MA–PbI 3 reported in ref. 17 . The initial coordinates of the molecular cations were chosen in such a way that the centre of mass is located in the middle of the cuboctahedral cavity, and the orientation of the four inequivalent cations in one unit cell follows the symmetry properties of the Pnma space group. Given the complexity of the total energy landscape of these systems, we checked the sensitivity of the structure with respect to the choice of the initial configuration in the case of NH 4 PbI 3 . This compound lies close to the stability limit ( Fig. 4b ), and can form quasi-1D structures in the presence of water [55] , [56] . In this case we performed structural optimizations using three additional initial configurations: (i) α a = α e =0, (ii) α a =0 and α e ≠0 with octahedra in phase along the apical direction, (iii) same as in (ii) but with octahedra out of phase. The optimized structures are all 3D perovskites, with total energy differences within 6 meV per atom. The largest deviation from the band gap reported in Fig. 3c is of 0.2 eV, and reflects the differences in the bond angles, following the trend predicted by the Platonic model in Fig. 2 . In the case of MA–PbI 3 it has been established that the spin–orbit interaction tends to reduce the scalar-relativistic band gap by ~1–1.1 eV (refs 20 , 22 ). This is consistent with our results shown in Fig. 3b . On the other hand, GW quasiparticle corrections do increase the value of the band gap [22] . Given these compensating corrections, and the fact that the very small relativistic band gaps are likely to induce significant errors in the calculation of the screened Coulomb interaction W , it is sensible to take scalar-relativistic calculations as the most consistent and unambiguous way to capture trends and identify the most promising structures. In order to check that the band gap trend obtained with DFT/LDA holds when using a higher level theory, we performed G 0 W 0 calculations using the Yambo code [57] for a few selected structures, namely AsH 4 PbI 3 , CH 3 NH 3 PbI 3 , CsPbI 3 and LiPbI 3 . For these calculations we used LDA norm conserving fully relativistic pseudopotentials for Pb and I, with semicore 5 d states included for Pb. The Kohn–Sham eigenfunctions and eigenvalues were calculated using a 100-Ry kinetic energy cutoff for all structures except LiPbI 3 , for which we used a cutoff of 130 Ry. The exchange and the correlation parts of the GW self-energy were calculated using planewaves cutoffs of 13 and 5 Ry, respectively (this is at the limit of what we can afford given the large unit cells). The screened Coulomb interaction W was described by means of the Godby–Needs plasmon-pole model [58] , and 400 bands were included in the sum over virtual states. The wavevector dependence of the screened Coulomb interaction was described by sampling the Brillouin zone using a Γ-centred 2 × 2 × 2 grid. A detailed discussion of these calculation is given in Supplementary Note 2 . Exciton-binding energy In order to estimate the magnitude of excitonic effects on the band gaps we calculate the exciton-binding energies using a simple Wannier exciton model [59] . In the Wannier model the exciton-binding energy is given by , where E 1 s is the energy of the fundamental state of the hydrogen atom, μ * is the effective mass of electrons and holes (that is, 1/ μ *=1/ m e +1/ m h ) and ε 0 the static (electronic) dielectric constant of the solid. This model is very approximate but should provide a fair representation of the trends in exciton-binding energies in our compounds. We calculated the effective mass tensors by approximating the second derivatives of the relativistic Kohn–Sham eigenvalues via finite differences, and taking the isotropic average in each case. Supplementary Fig. 2a,b shows the hole and electron effective masses thus obtained for the Platonic perovskite model, as a function of equatorial and apical metal–halide–metal bond angles. Our calculated effective masses are in line with previous calculations for CH 3 NH 3 PbI 3 and CsPbI 3 (refs 20 , 21 , 22 ). For the dielectric constant we performed finite-electric field calculations using the Berry-phase technique [60] , [61] . In this case we adopted a Γ-centred 2 × 2 × 4 Brillouin-zone mesh, with a finite electric field of 0.001 a.u. directed along the c axis. While in this case we did not not evaluate the isotropic average (purely in order to contain computational costs), Supplementary Figure 2d shows that this should not pose a problem since ε 0 does not depend strongly on the bond angles in the range of interest ( ε 0 =5.5–6.0). Platonic model of metal–halide perovskites Our ideal model of ABX 3 metal–organic halide perovskites consists of four inequivalent BX 6 Platonic octahedra in an orthorombic unit cell [17] , in absence of the cation. The octahedra are labelled O 1 –O 4 , as indicated in Fig. 1d , and are connected in a corner-sharing configuration. The B atoms occupy the centres of the octahedra, the X atoms are located at the corners and the metal–halide B–X distance is denoted by d . We set the origin of the reference frame at the centre of the octahedron O 1 , with its axes along the primitive vectors of the crystal lattice. The centres of the remaining three octahedra O 2 –O 4 are denoted by ( x , y ,0), (0,0, z ) and ( x , y , z ), respectively. The coordinates x , y and z will be determined below starting from the Euler angles described in the main text. The lattice parameters are expressed in terms of the centres of the octahedra as a =2 x , b =2 y and c =2 z . The corners of the octhedra are labelled as , with the superscript j identifying the octahedron, and the subscript i identifying a corner of the octahedron, as shown in Fig. 1c . The coordinates of each corner are referred to as . Octahedron O 1 . We consider an initial configuration where the octahedron O 1 has its apical diagonal along the c axis, and its equatorial edges along the a and b axes. The coordinates of the corners , and are by , and (0,0,1) d , respectively, while , and are obtained from these by changing the sign of all coordinates. In order to generate the most general structural models we perform a rotation of O 1 according to the three Euler angles , θ and φ . These angles define a sequence of spin, tilt and precession around the c axis. The tilt θ is performed via a rotation around a . This is illustrated in Fig. 1c . Following ref. 30 the matrix defining the rotation of the octahedron is: By applying this rotation to the initial coordinates of O 1 we obtain the position of the corners ( i =1,…,6) in their final orientation. These new coordinates are used to locate the centres and orientation of the remaining three octahedra. Octahedron O 2 . In order to determine the centre ( x , y , 0) of the octahedron O 2 we use the following observations: O 1 shares the corner with O 2 , and the corner with O 2′ , the periodic replica of O 2 along the a axis. Furthermore, O 2 shares the corner with O 1′ , the periodic replica of O 1 along the b axis. By requesting that the distance between the centre (C i ) of each octahedron and each corner is d in all cases, and that O 2 and O 2′ are both regular, we obtain the following equations relating the centre of O 2 with the position of the corner : After expressing the coordinates of in terms of the Euler angles , θ , and φ , we find that the above relations are verified simultaneously only when the spinning angle vanishes, . In this case the coordinates of the centre of O 2 are given by , and the coordinates of its corners are determined using the condition that the octahedron be regular. The explicit expressions for the coordinates of O 2 in terms of the corners of O 1 are: where the auxiliary variables p , q , r are given by: From the location of O 2 we can also determine the lattice parameters: , and c =4 d cos θ , where the last equation follows simply from the common tilt angle of O 1 and O 2 and the fact that they represent half of the unit cell along the c axis. In the case of vanishing tilt angle, θ =0, the spinning angle and the precession angle identify the same rotation, hence their distinction is not meaningful. In this case the relevant parameter appearing in all the equations is their sum . For consistency with the above rule that whenever θ ≠0, we here adopt the convention that always. In this case, when θ =0 the only other independent parameter is the precession angle φ . Obviously, this choice does not affect our results in any way. Octahedra O 3 and O 4 . From Fig. 1d we see that octahedron O 3 shares the corner with O 1 . As a consequence we have that octahedra O 3 and O 4 are centred at the positions 2 d (0,0,cos θ ) and , respectively. The corners of these octahedra are readily obtained by taking into account their regularity and the corner-sharing connectivity between O 3 and O 4 and between O 2 and O 4 . From the relations stated here it is clear that a cubic perovskite is obtained in the special case θ = φ =0. Furthermore, when the tilt angle vanishes, θ =0, we obtain two inequivalent tetragonal structures with identical lattice parameters. These structures correspond to the situations where the spinning angles of neighbouring octahedra along the apical direction are in-phase (same magnitude and same sign) or out-of-phase (same magnitude but different sign). As a general remark, the fact that the structure of the Platonic model is completely defined once we specify the values of two angles and the B–X bond length is quite remarkable. This property simplifies considerably the task of rationalizing the physics of metal–organic halide perovskites. Furthermore, the model illustrated here carries general validity and it can easily be adapted to describe other idealized perovskite structures. Apical and equatorial bond angles . The Euler angles θ and φ can be related to the intrinsic B–X–B bond angles. To this end we observe in Fig. 1d that α e is the angle between O 1 and O 2 through the corner , and α a is the angle between O 1 and O 3 through . Using the coordinates of the centres of O 1 –O 3 and the corners and determined as above, we find immediately cos α a =1−2cos 2 θ and cos α e =1−cos 2 φ (1+cos 2 θ ). Since cos 2 ( φ )≤1, the last two relations can be combined to yield the constraint cos( π − α a )≥2cos( π − α e )−1. For all the angles considered in Fig. 2 , the expansion of this inequality to first order in the angles is accurate to within 3% and reads . As a result, the Platonic model does not admit solutions with continuous corner-sharing connectivity in a region of the map bound by a straight line, as can be seen in Fig. 2 . Tolerance factor The Goldschmidt tolerance factor is given by , with R A , R B and R X the ionic radii of the elements in ABX 3 perovskites [42] . It was found empirically that 3D perovskite form when t is in the range 0.7–1.1 (refs 33 , 42 , 43 , 44 ). The lower bound corresponds to a situation where the cation is close enough to the halogen component to form a bond, thereby preventing the formation of a perovskite structure. The upper bound describes the case of the close-packed cubic perovskite structure. For values of t larger than 1 the perovskite structure is expected to distort or even form a layered perovskite structure [62] . For each structure we evaluated the Goldschmidt tolerance factor by using the steric sizes calculated via the DFT electron density and reported in Supplementary Table 1 . Material synthesis and characterization Perovskite precursor preparation . APbI 3 precursors were prepared by dissolving equimolar amounts of AI (where A=Li, Na, K, Rb and Cs) and PbI 2 in N,N-dimethylformamide at 0.5 M, in a nitrogen-filled glovebox. Mixtures were made by simply mixing the prepared precursors in the desired ratio. Film formation. Glass substrates were cleaned with acetone, isopropanol and oxygen plasma treatment. Thin films were formed by spin-coating on the substrates at 2,000 r.p.m. in the glovebox, and subsequently annealed on a hotplate by increasing the temperature until the formation of the dark phase was observed. This occurred at ~400 °C for CsPbI 3 and even higher for the Cs/Rb mixtures discussed in the main text. The 11% Rb film changed colour at 420 °C and the 20% Rb film at 470 °C. Optical measurements. Absorbance spectra were collected with a Varian Cary 300 UV–vis spectrophotometer with an internally coupled integrating sphere. How to cite this article : Filip, M. R. et al. Steric engineering of metal-halide perovskites with tunable optical band gaps. Nat. Commun. 5:5757 doi: 10.1038/ncomms6757 (2014).